Metallosupramolecular self-assembly of a universal 3-ravel In the realm of supramolecular chemistry, a small number of intricately interwoven structures that bridge the boundaries between art and science have been reported. These motifs, which typically form on the nanometre scale, display both considerable beauty and complexity. However, the generation of new topologies of this type has remained a very significant synthetic challenge. Here, we describe the synthesis of a discrete highly intertwined metallosupramolecular assembly based on a universal 3-ravel motif—a topology as yet unprecedented in supramolecular chemistry. The exotic, 20-component, [Fe 8 L 12 ] ravel entanglement may be considered as a 'branched knot', with individual molecules displaying either left- or right-handed chirality. The formation of this cluster was demonstrated by single-crystal and powder X-ray diffraction. The arrangement is stabilized by a favourable combination of π–π interactions and Nature's tendency to minimize voids in molecular architectures. Throughout human history aesthetically pleasing objects and structures have been admired as art, architecture or simply as attractive ornamental designs. In contrast, it is only since the rise of modern chemistry that it has become increasingly possible to parallel this aspect of the macro-world by constructing intricate structures and designs at the molecular level—in a few instances corresponding to attractive motifs that are not without artistic nuances. For example, over the past few decades considerable progress has been made in generating intertwined topologies [1] , [2] , [3] that include molecular trefoil knots [4] , Borromean rings [5] , [6] , Solomon knots [6] and mechanically interlinked structures of the catenane and rotaxane type [4] . Such intriguing architectures have been achieved using a variety of strategies, often involving significant practical and intellectual challenges, that are typically based on either metal template control or on the use of non-covalent interactions to direct the assembly process [4] , [7] . In particular instances structures of this type have also inspired the construction of simple molecular machines [8] , [9] , [10] . In recent work, our group has used aryl-linked bis-β-diketone or bis-β,δ-triketone ligands as self-assembling motifs for the synthesis of assorted metallocycles, helicates and cages along with a range of metal-organic frameworks [11] , [12] , [13] , [14] , [15] . We now describe the synthesis of a new bis-β-diketone derivative LH 2 incorporating a flexible oxy-bisphenylene linkage between the β-diketone domains (replacing the rigid phenylene or biphenylene spacers used in our previous studies). We also report the results of an investigation of its use for constructing new metal-containing supramolecular architectures. The introduction of limited flexibility into supramolecular building blocks, although tending to reduce the predictability of the resulting assemblies, can nevertheless result in the generation of new molecular topologies that are not able to be achieved without such flexibility [16] . Indeed, the interaction of LH 2 with ferric chloride generates a discrete highly intertwined metallosupramolecular assembly based on a universal 3-ravel motif ( Fig. 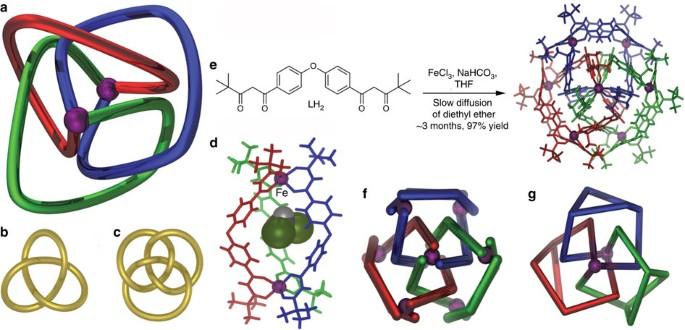Figure 1: Details of the universal 3-ravel and triple helicate structures. (a) Schematic representation of the universal 3-ravel topology; equivalent 'strands' are shown in different colours to aid visualization of the crossing points; purple balls highlight the nodes where the three strands meet. For comparison, representations of two other intertwined motifs: a trefoil knot,b, and Borromean rings,c, are presented. (d) X-ray structure of the uncharged dinuclear iron(III) triple helicate showing the included dichloromethane molecule in a space-filling representation; the highest occupancy positions of disordered components are shown. (e) Preparation and crystal structure of the 3-ravel together with two schematics,fandg, illustrating the ravel connectivity. 1a )—a molecular architecture so far unprecedented in supramolecular chemistry; trefoil knot and Borromean rings topologies are also illustrated in Figure 1b,c for comparison. The ravel terminology was first proposed in 2008, with individual ravel types (including, for example, universal 4-ravels) being predicted as possible exotic entanglement modes for both finite and infinite molecular systems [17] . The present 20-component, [Fe 8 L 12 ] ravel entanglement corresponds to a 'branched knot' topology, with individual molecules displaying chirality. The unique self-interpenetrating molecular arrangement is stabilized by a favourable combination of π–π interactions and Nature's tendency to minimize voids in molecular architectures. Figure 1: Details of the universal 3-ravel and triple helicate structures. ( a ) Schematic representation of the universal 3-ravel topology; equivalent 'strands' are shown in different colours to aid visualization of the crossing points; purple balls highlight the nodes where the three strands meet. For comparison, representations of two other intertwined motifs: a trefoil knot, b , and Borromean rings, c , are presented. ( d ) X-ray structure of the uncharged dinuclear iron(III) triple helicate showing the included dichloromethane molecule in a space-filling representation; the highest occupancy positions of disordered components are shown. ( e ) Preparation and crystal structure of the 3-ravel together with two schematics, f and g , illustrating the ravel connectivity. Full size image Ligand synthesis The ligand, 1,1′-(oxybis(1,4-phenylene))bis-4,4-dimethylpentance-1,3,-dione (LH 2 ), was synthesized in 81% yield by a Claisen condensation reaction. The peak at 16.05 p.p.m. in the 1 H nuclear magnetic resonance (NMR) spectrum indicates the ligand exists exclusively in its bis-enol form in chloroform solution. Triple helicate [dichloromethane ⊂ Fe 2 L 3 ] and universal 3-ravel [Fe 8 L 12 ] In an initial experiment, the reaction of LH 2 with ferric chloride in tetrahydrofuran (THF) in the presence of base yielded a deep-red solution that was taken to dryness and the red product recrystallized from a dichloromethane/ethanol mixture. The resulting soluble needle-like crystals (isolated in 88% yield) were used for an X-ray structure determination and shown to be a triple helicate of type [Fe 2 L 3 ] ( Fig. 1d ). The structure revealed that the helicate encapsulates a dichloromethane molecule in its central cavity; this guest is readily lost in a vacuum. Single crystals contain equal amounts of the P and M helical forms. If instead, diethyl ether vapour was very slowly diffused into the deep-red solution and the resulting mixture allowed to stand for ~3 months in a sealed flask, deep-red block-like crystals were obtained. Microanalysis of the vacuum dried crystals showed them to have an identical empirical composition to that of the above triple helicate product, but both the crystal habit and the solubility differed (unlike the triple helicate, the latter crystals were insoluble in common laboratory solvents). The yield was near quantitative at 97%. An X-ray structure determination showed that the latter product was an iron(III) cluster of type [Fe 8 L 12 ] whose structure ( Fig. 1e–g ) was characterized by an extraordinary 'self-interpenetrating' arrangement whose connectivity ascribes the universal 3-ravel motif. Comparison of the habits of the bulk crystalline products from the helicate and 3-ravel preparations, as well as comparison of their respective powder X-ray diffraction (PXRD) patterns (which also corresponded to those calculated from the respective corresponding single-crystal X-ray data, Fig. 2 ), confirmed the homogeneity of each product and that the crystal structures are truly representative of the bulk materials. 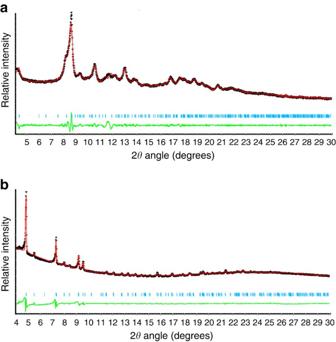Figure 2: The powder X-ray diffraction study. (a) X-ray powder diffraction pattern of [DCM⊂Fe2L3]. The black crosses show the collected data, the red line the calculated Le Bail fit, the green line the difference plot and the vertical blue lines the reflection markers. Modelled using space group no. 61,Pbca,a=21.625(2),b=19.443(1),c=41.085(4) Å.Rp=1.601%,Rwp=2.416%,χ2=3.252%. (b) Powder X-ray diffraction pattern of [Fe8L12]·15Et2O. The black crosses show the collected data, the red line the calculated Le Bail fit, the green line the difference plot and the vertical blue lines the reflection markers. Modelled using space group no. 163,P1c,a=31.968(5),c=24.079(4) Å.Rp=1.644%,Rwp=2.578%,χ2=36.705%. Figure 2: The powder X-ray diffraction study. ( a ) X-ray powder diffraction pattern of [DCM ⊂ Fe 2 L 3 ]. The black crosses show the collected data, the red line the calculated Le Bail fit, the green line the difference plot and the vertical blue lines the reflection markers. Modelled using space group no. 61, Pbca , a =21.625(2), b =19.443(1), c =41.085(4) Å. R p =1.601%, R wp =2.416%, χ 2 =3.252%. ( b ) Powder X-ray diffraction pattern of [Fe 8 L 12 ]·15Et 2 O. The black crosses show the collected data, the red line the calculated Le Bail fit, the green line the difference plot and the vertical blue lines the reflection markers. Modelled using space group no. 163, P 1 c, a =31.968(5), c =24.079(4) Å. R p =1.644%, R wp =2.578%, χ 2 =36.705%. Full size image The unique D 3 -symmetric universal 3-ravel is derived from 20 individual components (12 ligands and 8 metal ions) and very likely represents the thermodynamic product from the reaction of these components given the extended time required for this interwoven topology to form. Each molecule of the ravel is associated with a helical twist, with all eight iron atoms adopting the same chiral configuration; hence, single molecules are chiral, whereas individual crystals are racemic, containing equal numbers of opposite chiral forms. Interpenetration of porous polymeric structures is common in the crystalline state, with the driving force usually attributed to the achievement of less void volume in the crystal—in keeping with Aristotle's maxim that 'Nature abhors a vacuum'. In this context, examples of slow interpenetration (and linking) of molecular cages by reversible metal coordination bond formation have been documented previously [18] , [19] , [20] and, for example, Fujita et al . have pointed out that interlocked cage structures can be more stable than their separated monomer units [18] . Quite recently, interpenetration by slow reversible covalent (imine) bond formation has also been shown to give rise to an organic interlocked cage structure [21] , [22] . Although non-covalent interactions such as π–π stacking undoubtedly contribute to stabilization of this product in the solid state, it has been suggested [22] that the generation of a more compact, interpenetrated assembly provides an additional driving force for the formation of the interlocked product in this case. The operation of a related interpenetration mechanism seems to be a reasonable rationale for promoting the intertwining found in the present [Fe 8 L 12 ] assembly. The adoption of the universal 3-ravel topology clearly provides an efficient means of 'space filling' to produce what, overall, is a quite compact molecular arrangement ( Fig. 3a ). In addition, in the solid state, there is evidence for favourable π–π stacking between aryl rings and these interactions presumably act in concert with the above mechanism to direct the ravel assembly process and stabilize the final product; related π–π stacking is absent in the isomeric [Fe 2 L 3 ] helicate structure shown in Figure 2 . 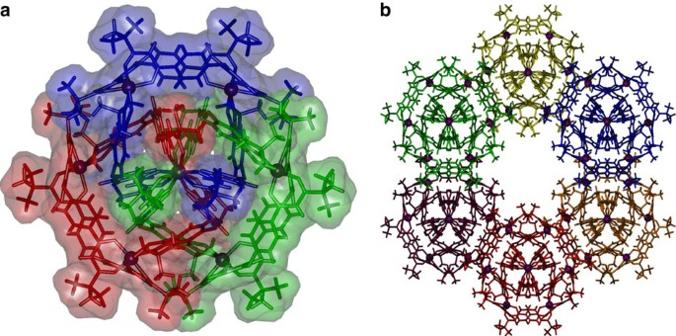Figure 3: The universal 3-ravel structure. (a) Semi-transparent space-filling representation of the X-ray structure of the universal 3-ravel, [Fe8L12] showing the 'close packing' of the ravel strands. (b) Schematic representation of part of the crystal packing of [Fe8L12] showing the top of one of the one-dimensional channels present in the crystal structure; solvate molecules have been omitted for clarity. A view of the crystal packing is given in Figure 3b . Figure 3: The universal 3-ravel structure. ( a ) Semi-transparent space-filling representation of the X-ray structure of the universal 3-ravel, [Fe 8 L 12 ] showing the 'close packing' of the ravel strands. ( b ) Schematic representation of part of the crystal packing of [Fe 8 L 12 ] showing the top of one of the one-dimensional channels present in the crystal structure; solvate molecules have been omitted for clarity. Full size image In this report, we describe the realization of a new class of interwoven molecular nanostructures based on a universal 3-ravel motif. The resulting tightly organized iron(III) nanocluster spontaneously assembles over time from 8 iron and 12 bis-β-diketonato ligand components. The formation of this unique self-interpenetrating molecular arrangement appears, at least in part, to be driven by Nature's tendency to minimize voids in molecular architectures. Finally, it is noted that the present ravel structure exhibits both remarkable intricacy and unusual beauty in its molecular form, it thus provides a new member of the small family of diverse interwoven molecular architectures displaying similar attributes reported previously. Physical measurements 1 H- and 13 C-NMR spectra were recorded on a Bruker 300 MHz spectrometer (Bruker) at 300 K. The electron spray mass spectra were obtained with a Bruker Daltonics Apex Ultra 7T FTICR mass spectrometer (Bruker) with an electrospray ionization source. Elemental analyses for C, H and N were performed by Campbell Microanalytical Laboratory, University of Otago. Infrared spectra were recorded on a Varian 800 Fourier transform infrared spectrometer (Varian) as KBr pellets. Preparation of LH 2 3,3-Dimethyl-2-butanone (2.1 g, 21.0 mmol) in THF (100 ml) was added dropwise to a stirred suspension of NaH (2.5 g, 63.0 mmol, 60% oil dispersion) in THF (150 ml) under nitrogen at room temperature. After 10 min the resulting mixture was treated with a solution of 4,4′-oxybis(methyl benzoate) (3.0 g, 10.5 mmol) in THF (100 ml), which was added dropwise over 20 min. The mixture was heated at reflux overnight during which time it slowly turned yellow. The solution was allowed to cool and the solvent was removed. The yellow residue was dissolved in ice water (200 ml), the solution was filtered and diethyl ether (60 ml) was added to the filtrate and the mixture was shaken. The aqueous phase was separated then acidified using dilute hydrochloric acid to yield a precipitate. This mixture was allowed to stand for 1 h in an ice bath and the precipitate was collected by filtration and recrystallized from an acetone/ethanol mixture to yield colourless needles. Yield: 3.6 g (81%), m.p. : 108–110 °C; 1 H NMR (300 MHz, CDCl 3 ): δ 16.55 (brs, 2H, O H ), 7.91 (d, J =8.8 Hz, 4H, Ar-C H ), 7.08 (d, J =8.8 Hz, 4H, Ar-C H ), 6.26 (s, 2H, =C H ), 1.25 (s, 18H, C H 3 ); 13 C NMR (300 MHz, CDCl 3 ): δ 202.05, 184.28, 159.69, 131.30, 129.23, 118.87, 91.69, 39.68, 27.45; IR (KBr pellets): 2974, 2869, 1596, 1506, 1459, 1290, 1261, 1166, 847, 792 cm −1 ; HRMS (CH 3 OH/DCM, m/z ): [M+H] + calcd for C 26 H 31 O 5 , 423.21660; found, 423.21671; analysis (calcd, found for C 26 H 30 O 5 ): C (73.90, 73.83), H (7.16, 7.39). Preparation of [Fe 2 L 3 ] LH 2 (100 mg, 0.24 mmol) in dry THF (40 ml) was added to NaHCO 3 , (1.0 g, 0.012 mol) in dry THF (10 ml). The mixture was stirred for 1 h before anhydrous iron(III) chloride (26 mg, 0.16 mmol) dissolved in dry THF (40 ml) was added dropwise. The mixture was stirred overnight, during which time the colour changed to deep-red. The mixture was filtered and the filtrate was collected. The solvent was removed on a rotary evaporator and the crude solid obtained was recrystallized from DCM/ethanol (V:V=1:1). Yield: 97 mg (88%). A red needle from the solution was used directly for the X-ray structure determination. Analysis (calcd, found for C 78 H 84 Fe 2 O 15 ): C (68.20, 68.17), H (6.17, 6.18). Preparation of [Fe 8 L 12 ] LH 2 (100 mg, 0.24 mmol) in dry THF (40 ml) was added to NaHCO 3 , (1.0 g, 0.012 mol) in dry THF (10 ml). The mixture was stirred for 1 h before anhydrous iron(III) chloride (26 mg, 0.16 mmol) dissolved in dry THF (40 ml) was added dropwise. The mixture was stirred overnight, during which time the colour changed to deep-red. The mixture was filtered and the filtrate was collected. The large red block crystals were formed by the very slow diffusion of diethyl ether into this resulting solution over ~3 months. Yield: 107 mg (97%). A crystal from this solution was used directly for the X-ray structure determination. Analysis (calcd, found for C 312 H 336 Fe 8 O 60 ): C (68.20, 67.80), H (6.17, 6.37). Single-crystal X-ray diffraction measurements X-ray structural data were collected on a Bruker-Nonius APEX2-X8-FR591 diffractometer (Bruker-Nonius) using graphite-monochromated MoKα radiation generated from a rotating anode (0.71073 Å) with ω and ϕ scans at 150 K (ref. 23 ). Multi-scan empirical absorption corrections were applied using the programme SADABS [24] . Data integration and reduction were undertaken with SAINT and XPREP [23] and subsequent computations were carried out using the WinGX-32 and XSEED graphical user interfaces [25] , [26] . The structures were solved by direct methods using SHELXS-97 or SIR97 (refs 27 , 28 ). Data were refined and extended with SHELXL-97 (ref. 29 ). Non-hydrogen atoms were refined anisotropically. Carbon-bound hydrogen atoms were included in idealized positions and refined using a riding model. The crystals used in the study were unstable (rapid solvent loss) and in both cases rapid mounting (<1 min) at 200 K before quenching in the cryostream was required to enable data collection. Disorder, where present, was modelled with standard crystallographic techniques, including the use of bond length and angle restraints where required. Specific refinement details for each structure are given below. [DCM ⊂ Fe 2 L 3 ] Formula C 79 H 86 Cl 2 Fe 2 O 15 , M 1458.08, orthorhombic, space group P bca(#61), a 21.757(2), b 16.820(2), c 41.600(3) Å, V 15224(3) Å 3 , D c 1.272 g cm −3 , Z 8, crystal size 0.15×0.10×0.05 mm 3 , colour orange, habit needle, temperature 150(2) K, λ (MoKα) 0.71073 Å, μ (MoKα) 0.514 mm −1 , T (SADABS) min,max 0.824693, 1.00000, 2 θ max 41.62, hkl range −21 21, −16 16, −41 31, N 42805, N ind 7950( R merge 0.1049), N obs 4792(I > 2 σ (I)), N var 919, residuals * R 1( F ) 0.0543, wR 2( F 2 ) 0.1476, GoF(all) 1.005, Δ ρ min,max −0.890, 0.659 e − Å −3 . * R 1=Σ|| F o | - | F c ||/Σ| F o | for F o > 2 σ ( F o ); wR 2=(Σw( F o 2 – F c 2 ) 2 ) 1/2 /Σ(w F c 2 ) 2 ) 1/2 all reflections w =1/[ σ 2 ( F o 2 )+(0.0746 P ) 2 +9.8604 P ] where P =( F o 2 +2 F c 2 )/3. The crystals used in the study were small and poorly diffracting. In addition, they decayed quickly out of solvent and rapid handling was required. Combined, this resulted in less than ideal data (high R int , low completeness and low redundancy) with very few reflections observed at >50° 2 θ . Nevertheless, the quality of the data is more than sufficient for establishing the connectivity of the structure. The encapsulated dichloromethane molecule and the C(74) containing tertiary butyl group are disordered over three positions of occupancies 0.5, 0.25 and 0.25. Each of the disordered non-hydrogen atoms in these groups was modelled with identical thermal parameters. [Fe 8 L 12 ]·15Et 2 O Formula C 372 H 486 Fe 8 O 75 , M 6604.41, trigonal, space group P 1 c(#163), a 31.3870(10), b 31.3870(10), c 25.222(2) Å, γ 120.00°, V 21518(2) Å 3 , D c 1.019 g cm −3 , Z 2, crystal size 0.53×0.39×0.35 mm 3 , colour red, habit block, temperature 150(2) K, λ (MoKα) 0.71073 Å, μ (MoKα) 0.325 mm −1 , T (SADABS) min,max 0.6359, 0.7450, 2 θ max 44.98, hkl range −33 33, −33 33, −23 27, N 77748, N nd 9355( R merge 0.0479), N obs 5850(I > 2 σ (I)), N var 607, residuals * R 1( F ) 0.0954, wR 2( F 2 ) 0.2992, GoF(all) 1.116, Δ ρ min,mas −0.836, 1.357 e − Å −3 . * R 1=Σ|| F o| − | F c||/Σ| F o| for F o > 2 σ ( F o); wR 2=(Σ w ( F o 2 – F c 2 ) 2 ) 1/2 all reflections w =1/[ σ 2 ( F o 2 )+(0.2000 P ) 2 +0.0000 P ] where P =( F o 2 +2 F c 2 )/3. The crystals used in this study decayed extremely rapidly out of solvent. Despite rapid handling at dry-ice temperatures (<1 min), quenching in the nitrogen cryostream, long exposure times and the use of a high-power laboratory source (5 kW from a rotating anode), the data were less than ideal with only reflections to ~1.0 Å resolution being recorded. Nevertheless, the data is more than adequate to confirm connectivity. These difficulties are associated with the unit cell containing substantial voids and a large amount of disordered solvent (diethyl ether). The SQUEEZE function of PLATON [30] was used to remove the contribution of these molecules to the data. In addition to the presence of substantial disordered solvent, each of the tertiary butyl groups on the exterior of the molecule (that is all except that containing C (49)) is disordered and was modelled over multiple positions with a total occupancy of one in each case. A number of constraints and restraints were required in these regions to facilitate realistic modelling. The Cambridge Crystallographic Data Centre (http:// www.ccdc.cam.ac.uk/conts/retrieving.html ) hosts the crystallographic data for these compounds. Deposition numbers: CCDC-791998 and CCDC-791999. Details are given in Supplementary Data 1 and Supplementary Data 2 . PXRD measurements PXRD measurements were collected using a PANalytical X'Pert PRO MPD X-ray diffractometer equipped with a PIXcel detector and using Cu kα radiation (λ av. =1.5419 Å). The [Fe 2 L 3 ] sample was measured with the diffractometer set up in Bragg PDS mode using a spinning flat plate holder. The [Fe 8 L 12 ] sample was measured using the diffractometer in capillary mode with a 0.3 mm ID glass capillary into which the sample and solvent were sealed. Data were collected from 4–30° (2 θ ) using a step size of 0.013° (2 θ ) and a counting time of 99 s ([Fe 2 L 3 ])/6,437 s ([Fe 8 L 12 ]) with the PIXcel detector in scanning mode (active length 3.35°) giving 18,669 counts [Fe 2 L 3 ]/244,980 counts [Fe 8 L 12 ] for the most intense peak. Data analysis was performed using the Le Bail method [31] as implemented in the Rietica software package [32] using a Pseudo-Voigt (Howard asymmetry.) peak shape model and automatic background smoothing function for the [Fe 2 L 3 ] sample and a shifted Chebyshev II polynomial with six terms for the [Fe 8 L 12 ] background. The refined patterns for [Fe 2 L 3 ] and [Fe 8 L 12 ] are given in Figure 2 . The χ 2 value for [Fe 8 L 12 ] (36.705%) is unusually large because of the higher than normal background contribution resulting from the spinning glass capillary. Despite the difficulty in modelling the background model represents a good fit to the data ( R p =1.644%, R wp =2.578%) with only a small amount of peak mismatch at ~4.5°. How to cite this article: Li, F. et al . Metallosupramolecular self-assembly of a universal 3-ravel. Nat. Commun. 2:205 doi: 10.1038/ncomms1208 (2011).